A truncated Wnt7a retains full biological activity in skeletal muscle Wnt signaling has essential roles during embryonic development and tissue homoeostasis. Wnt proteins are post-translationally modified and the attachment of a palmitate moiety at two conserved residues is believed to be a prerequisite for the secretion and function of Wnt proteins. Here we demonstrate that a mammalian Wnt protein can be fully functional without palmitoylation. We generate a truncated Wnt7a variant, consisting of the C-terminal 137 amino acids lacking the conserved palmitoylation sites and show that it retains full biological activity in skeletal muscle. This includes binding to and signaling through its receptor Fzd7 to stimulate symmetric expansion of satellite stem cells by activating the planar-cell polarity pathway and inducing myofibre hypertrophy by signaling through the AKT/mTOR pathway. Furthermore, this truncated Wnt7a shows enhanced secretion and dispersion compared with the full-length protein. Together, these findings open important new avenues for the development of Wnt7a as a treatment for muscle-wasting diseases and have broad implications for the therapeutic use of Wnts as biologics. The Wnt family of genes encodes 19 cysteine-rich, secreted glycoproteins, which bind specific members of the Frizzled (Fzd) transmembrane receptor family on target cells [1] . All Wnt proteins share a signal sequence for secretion, several glycosylation sites and a characteristic distribution of 22 cysteine residues [2] , [3] . Wnts have essential roles as mediators of developmental processes in vertebrates and invertebrates [2] , and it has been suggested that palmitoylation is absolutely required for the efficient secretion and activity of Wnts [4] , [5] , [6] . Canonical Wnt signaling is characterized by the binding of Wnt proteins to Fzd receptors, thereby activating Dishevelled, which leads to the inactivation of the serine/threonine kinase glycogen synthase kinase-3beta (GSK3beta). Inhibition of GSK3beta results in the stabilization of beta-catenin. Non-canonical Wnt signaling can lead to the activation of Rho and JAK or stimulation of calcium influx and activation of PKC and CamKII independently of GSK3beta activation [2] . Recently, two additional non-canonical Wnt signaling pathways have been demonstrated to be active in skeletal muscle, both of which are mediated by Wnt7a and utilize Fzd7 as a membrane receptor. Wnt7a activates the planar-cell polarity pathway in satellite stem cells which drives their symmetric expansion [7] . In adult myofibres and myotubes, Wnt7a binds to Fzd7, in order to activate signaling through PI3kinase in a G-protein alpha S-dependent manner to stimulate the anabolic AKT/mTOR pathway resulting in the hypertrophy of myotubes and myofibres [8] . The primary amino-acid sequence of Wnt proteins predicts solubility in aqueous solution. However, Wnt proteins are strongly hydrophobic and are mostly found associated with the extracellular matrix (ECM) [9] . These observations led to the notion that Wnt proteins are modified post-translationally. Wnt proteins were indeed found to be subject to N-linked glycosylation during their biosynthesis [10] . Moreover, Wnt proteins are lipid-modified by the attachment of a palmitate moiety at two conserved residues [11] . Importantly, this palmitoylation has been suggested to be absolutely required for Wnt activity [4] , [5] , [6] . While this manuscript was in preparation, the structural basis of Wnt recognition by Fzd receptors was reported and this work suggested a two-domain structure of Wnt proteins, with one side being dominated by a palmitoleic acid group and the other one forming a hydrophobic amino-acid contact with the Fzd receptor [12] . To investigate whether palmitoylation of Wnt7a, one of the major Wnts involved in muscle regeneration, is a prerequisite for its function, we generated a truncated Wnt7a variant (Wnt7a-CT) consisting of the C-terminal 137 aa, which hence lacks both palmitoylation sites. Here we demonstrate that the Wnt7a-CT variant is active without palmitoylation and fully functional in skeletal muscle. These findings represent an important advance in the development of Wnt-based therapeutics. Wnt7a-CT induces hypertrophy in skeletal muscle We first asked whether Wnt7a-CT is able to induce hypertrophy in cultured myotubes. C2C12 myoblasts were transiently transfected with expression plasmids for full-length Wnt7a (Wnt7a-FL), Wnt7a-CT ( Fig. 1a ), or a control plasmid, and differentiated for 5 days. Myotubes expressing the Wnt7a-CT construct demonstrated robust hypertrophy and exhibited a 1.3-fold increase in the diameter that was similar to the level of hypertrophy induced by Wnt7a-FL (1.2-fold increase) ( Fig. 1b,c ). These findings suggest that the active domain of Wnt7a is localized in the C-terminal portion of the protein, and that palmitoylation is not a prerequisite for its function in cell culture. 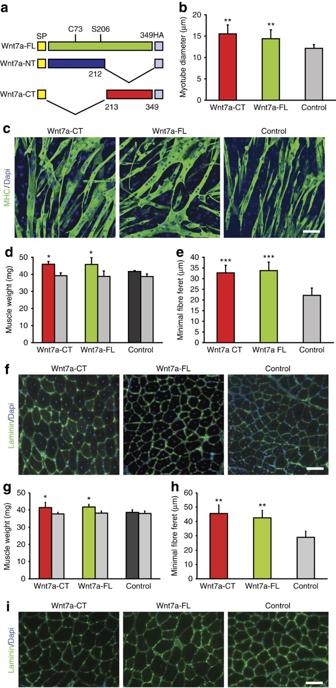Figure 1: Wnt7a-CT induces hypertrophy in differentiated myotubes and myofibres. (a) Schematic showing the different Wnt7a variants used. SP: signal peptide, the Wnt7a full-length (FL) protein is palmitoylated on C73 and S206. (b) C2C12 cells were transiently transfected with an expression plasmid for Wnt7a-CT, Wnt7a-FL or a control plasmid and differentiated for 5 days,n=4, **P<0.01. (c) C2C12 cells were transiently transfected with Wnt7a-CT, Wnt7a-FL or a control plasmid and differentiated for 5 days. Staining for MHC (myosin heavy chain, in green) marks differentiated cells, nuclei are counterstained with Dapi (in blue). Scale bar: 20 μm. (d) Electroporation of a Wnt7a-CT, Wnt7a-FL or control plasmid into the TA muscle of C57/BL6 mice resulted in increased muscle wet weight in muscles electroporated with the Wnt7a-CT and Wnt7a-FL plasmids 2 weeks after electroporation,n=4, *P<0.05. The weight of the contralateral leg is shown as grey bars. (e) Electroporation of the TA muscle with a Wnt7a-CT and a Wnt7a-FL expression plasmid resulted in increased fibre calibre,n=4, ***P<0.001. (f) Representative images of immunostained sections of TA muscles as indandefor laminin (in green); nuclei are counterstained with Dapi (in blue). Scale bar: 100 μm. (g) Injection of Wnt7a-CT or Wnt7a-FL protein into the TA muscle of C57/BL6 mice resulted in increased muscle wet weight in muscles 2 weeks after injection,n=4, *P<0.05. The weight of the contralateral leg is shown as grey bars. (h) Injection of the TA muscle with Wnt7a-CT and Wnt7a-FL proteins resulted in increased fibre calibre,n=4, **P<0.01. (i) Representative images of immunostained sections of TA muscles as ingandhfor laminin (in green); nuclei are counterstained with Dapi (in blue). Scale bar: 100 μm. AllP-values were calculated using a two-tailed Student’st-test. All data are expressed as mean±s.e.m. Figure 1: Wnt7a-CT induces hypertrophy in differentiated myotubes and myofibres. ( a ) Schematic showing the different Wnt7a variants used. SP: signal peptide, the Wnt7a full-length (FL) protein is palmitoylated on C73 and S206. ( b ) C2C12 cells were transiently transfected with an expression plasmid for Wnt7a-CT, Wnt7a-FL or a control plasmid and differentiated for 5 days, n =4, ** P <0.01. ( c ) C2C12 cells were transiently transfected with Wnt7a-CT, Wnt7a-FL or a control plasmid and differentiated for 5 days. Staining for MHC (myosin heavy chain, in green) marks differentiated cells, nuclei are counterstained with Dapi (in blue). Scale bar: 20 μm. ( d ) Electroporation of a Wnt7a-CT, Wnt7a-FL or control plasmid into the TA muscle of C57/BL6 mice resulted in increased muscle wet weight in muscles electroporated with the Wnt7a-CT and Wnt7a-FL plasmids 2 weeks after electroporation, n =4, * P <0.05. The weight of the contralateral leg is shown as grey bars. ( e ) Electroporation of the TA muscle with a Wnt7a-CT and a Wnt7a-FL expression plasmid resulted in increased fibre calibre, n =4, *** P <0.001. ( f ) Representative images of immunostained sections of TA muscles as in d and e for laminin (in green); nuclei are counterstained with Dapi (in blue). Scale bar: 100 μm. ( g ) Injection of Wnt7a-CT or Wnt7a-FL protein into the TA muscle of C57/BL6 mice resulted in increased muscle wet weight in muscles 2 weeks after injection, n =4, * P <0.05. The weight of the contralateral leg is shown as grey bars. ( h ) Injection of the TA muscle with Wnt7a-CT and Wnt7a-FL proteins resulted in increased fibre calibre, n =4, ** P <0.01. ( i ) Representative images of immunostained sections of TA muscles as in g and h for laminin (in green); nuclei are counterstained with Dapi (in blue). Scale bar: 100 μm. All P -values were calculated using a two-tailed Student’s t -test. All data are expressed as mean±s.e.m. Full size image To confirm that Wnt7a-CT is acting extracellularly, we applied Wnt7a-CT or Wnt7a-FL-containing cell culture supernatant from COS cells or supernatant from COS cells transfected with a plasmid control on differentiated myotubes. Cells were collected 2 days later and the extent of hypertrophy was evaluated ( Fig. 2a,b ). Application of media containing Wnt7a-CT resulted in robust myotube hypertrophy (1.2-fold increase) as did the full-length protein Wnt7a-FL (1.3-fold increase). By using supernatant from COS cells transfected with a plasmid control, we excluded indirect effects from the cell culture media. 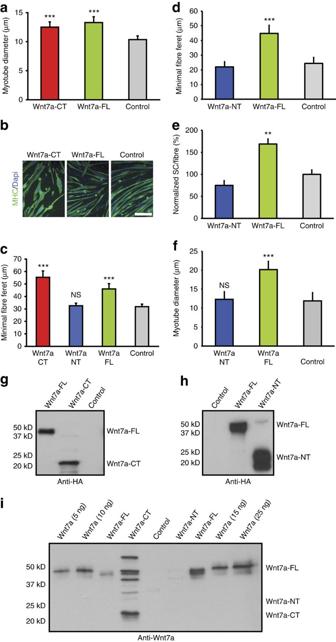Figure 2: Wnt7a-CT but not Wnt7a-NT induces hypertrophy. (a) C2C12 cells were incubated on day 3 of differentiation with Wnt7a-CT, Wnt7a-FL or a vehicle control. After 5 days of differentiation, the myotube diameter was assessed,n=4, ***P<0.001. (b) C2C12 cells were incubated with Wnt7a-CT, Wnt7a-FL or a control on day 3 of differentiation and differentiated for 2 additional days. Staining for MHC (myosin heavy chain, in green) marks differentiated cells; nuclei are counterstained with Dapi (in blue). Scale bar: 50 μm. (c) TA muscles from C57/BL6 mice were electroporated with expression plasmids for Wnt7a-CT, Wnt7a-NT, Wnt7a-FL or a control plasmid; the minimal fibre feret of electroporated fibres was assessed,n=4, ***P<0.001. (d) TA muscles from C57/BL6 mice were injected with Wnt7a-NT or Wnt7a-FL protein, and the minimal fibre feret was assessed,n=4, ***P<0.001. (e) Injection of Wnt7a-NT protein does not lead to increased numbers of Pax7-positive satellite cells,n=4, **P<0.01. (f) C2C12 cells were transiently transfected with Wnt7a-NT, Wnt7a-FL or a control plasmid,n=3, ***P<0.001. (g) Immunoblot analysis using antibodies directed against the HA-tag of the Wnt7a-CT and Wnt7a-FL proteins demonstrate that similar amounts of Wnt7a-CT and Wnt7a-FL proteins were purified. (h) Immunoblot analysis using antibodies directed against the HA-tag of the Wnt7a-NT and Wnt7a-FL proteins demonstrate that similar amounts of protein were purified. (i) Immunoblot analysis using antibodies directed against Wnt7a were used to determine the protein amounts injected into TA muscles. AllP-values were calculated using a two-tailed studentst-test. All data are expressed as mean±s.e.m. Figure 2: Wnt7a-CT but not Wnt7a-NT induces hypertrophy. ( a ) C2C12 cells were incubated on day 3 of differentiation with Wnt7a-CT, Wnt7a-FL or a vehicle control. After 5 days of differentiation, the myotube diameter was assessed, n =4, *** P <0.001. ( b ) C2C12 cells were incubated with Wnt7a-CT, Wnt7a-FL or a control on day 3 of differentiation and differentiated for 2 additional days. Staining for MHC (myosin heavy chain, in green) marks differentiated cells; nuclei are counterstained with Dapi (in blue). Scale bar: 50 μm. ( c ) TA muscles from C57/BL6 mice were electroporated with expression plasmids for Wnt7a-CT, Wnt7a-NT, Wnt7a-FL or a control plasmid; the minimal fibre feret of electroporated fibres was assessed, n =4, *** P <0.001. ( d ) TA muscles from C57/BL6 mice were injected with Wnt7a-NT or Wnt7a-FL protein, and the minimal fibre feret was assessed, n =4, *** P <0.001. ( e ) Injection of Wnt7a-NT protein does not lead to increased numbers of Pax7-positive satellite cells, n =4, ** P <0.01. ( f ) C2C12 cells were transiently transfected with Wnt7a-NT, Wnt7a-FL or a control plasmid, n =3, *** P <0.001. ( g ) Immunoblot analysis using antibodies directed against the HA-tag of the Wnt7a-CT and Wnt7a-FL proteins demonstrate that similar amounts of Wnt7a-CT and Wnt7a-FL proteins were purified. ( h ) Immunoblot analysis using antibodies directed against the HA-tag of the Wnt7a-NT and Wnt7a-FL proteins demonstrate that similar amounts of protein were purified. ( i ) Immunoblot analysis using antibodies directed against Wnt7a were used to determine the protein amounts injected into TA muscles. All P -values were calculated using a two-tailed students t -test. All data are expressed as mean±s.e.m. Full size image We previously demonstrated that a single injection of the full-length Wnt7a protein into the tibialis anterior (TA) muscle results in an efficient induction of hypertrophy [8] . To test whether the C-terminus of Wnt7a is also able to similarly induce hypertrophy in this context, we electroporated TA muscles from adult C57/BL6 mice with expression plasmids for Wnt7a-CT, Wnt7a-FL or a control plasmid. Muscles electroporated with either Wnt7a-CT or Wnt7a-FL expression plasmids demonstrated robust hypertrophy, resulting in increased muscle wet weights (10.2 or 9.9% increase) and increased minimal fibre feret (47.8% and 52.5% increase, respectively) relative to muscles electroporated with a control plasmid ( Fig. 1d–f ). Furthermore, we injected cell culture supernatant containing 150 ng of Wnt7a-CT or Wnt7a-FL protein into the TA muscle of C57/BL6 mice ( Fig. 2g,i ). A single injection leads to an increase in muscle wet weights by 7.3% and 8.2%, respectively ( Fig. 1g ) as well as an increase in fibre feret (57% and 47% increase, respectively, Fig. 1h,i ). To investigate the activity of the N-terminal portion of Wnt7a (1–212 aa), we electroporated expression plasmids for Wnt7a-NT, Wnt7a-CT or Wnt7a-FL versus a control plasmid into TA muscle ( Fig. 2c ). Importantly, only fibres electroporated with either the Wnt7a-FL or the Wnt7a-CT construct, were found to be hypertrophic (44.7 or 74.1% increase in the minimal fibre feret, respectively), suggesting that only Wnt7a-CT but not the Wnt7a-NT variant is capable of inducing hypertrophy. Moreover, we injected equal amounts of Wnt7a-NT or Wnt7a-FL protein-containing cell supernatant into the TA muscle of C57/BL6 mice ( Fig. 2h,i ). We observed that only the full-length protein but not the N-terminus of Wnt7a was able to induce hypertrophy ( Fig. 2d ), further supporting the notion that the active domain of Wnt7a is located in the C-terminus and not in the N-terminus. Furthermore, we transiently transfected C2C12 cells with the Wnt7a-NT plasmid and also found that in this context Wnt7a-NT was not able to induce hypertrophy. We have previously shown that Wnt7a induction of hypertrophy is dependent on the receptor Fzd7 [8] . To investigate whether Wnt7a-CT induces hypertrophy through the same receptor as the full-length protein, we used a small interfering RNA (siRNA)-mediated approach targeting Fzd7. Transfection of Fzd7 siRNA fully abrogated the ability of Wnt7a-CT and Wnt7a-FL to induce hypertrophy ( Fig. 3a , Supplementary Fig. S1 ). Thus, we conclude that Wnt7a-CT similarly signals through Fzd7. Moreover, we found that Wnt7a-CT activates the AKT/mTOR pathway ( Fig. 3b ), as evidenced by the increased phosphorylation of two core components of this pathway, AKT and S6. Furthermore, we demonstrated that expression of Wnt7a-CT stimulated increased levels of pAKT in myofibres in a manner identical to Wnt7a-FL ( Fig. 3d ). Interestingly, both Wnt7a-CT and Wnt7a-FL induced phosphorylation of AKT in fibres expressing Wnt7a-CT and Wnt7a-FL, as well as in the surrounding fibres. 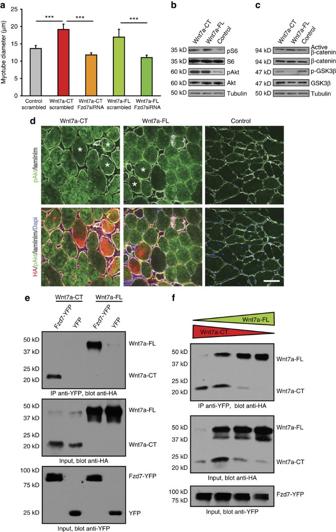Figure 3: Wnt7a-CT activates the AKT/mTOR pathway through binding to Fzd7. (a) siRNA-mediated knockdown of Fzd7 inhibited the induction of hypertrophy in Wnt7a-CT- and Wnt7a-FL-expressing myotubes,n=4, ***P<0.001. (b) Immunoblot analyses revealed increased levels of phosphorylation of members of the AKT/mTOR pathway in C2C12 myotubes expressing Wnt7a-CT or Wnt7a-FL compared with control cells. (c) Immunoblot analyses revealed no changes in the amount of phosphorylated or total GSK3beta and the amount of active beta-catenin or total beta-catenin in Wnt7a-CT expressing C2C12 myotubes compared with control cells, suggesting that neither Wnt7a-CT nor Wnt7a-FL act through the canonical Wnt pathway. (d) Electroporation of a Wnt7a-CT or Wnt7a-FL expression plasmid into the TA muscle of C57/BL6 mice resulted in increased levels of pAKT compared with muscles electroporated with a control plasmid. Staining for HA in red, pAKT in green, laminin in white, nuclei are counterstained with Dapi (in blue). Electroporated fibres are marked by an asterisk. Scale bar: 20 μm. (e) Co-immunoprecipitation analysis demonstrates that both Wnt7a-CT and Wnt7a-FL bind Fzd7-YFP. (f) Co-immunoprecipitation analysis suggests that Wnt7a-CT and Wnt7a-FL bind to Fzd7-YFP with similar affinity. AllP-values were calculated using a two-tailed Student’st-test. All data are expressed as mean±s.e.m. Figure 3: Wnt7a-CT activates the AKT/mTOR pathway through binding to Fzd7. ( a ) siRNA-mediated knockdown of Fzd7 inhibited the induction of hypertrophy in Wnt7a-CT- and Wnt7a-FL-expressing myotubes, n =4, *** P <0.001. ( b ) Immunoblot analyses revealed increased levels of phosphorylation of members of the AKT/mTOR pathway in C2C12 myotubes expressing Wnt7a-CT or Wnt7a-FL compared with control cells. ( c ) Immunoblot analyses revealed no changes in the amount of phosphorylated or total GSK3beta and the amount of active beta-catenin or total beta-catenin in Wnt7a-CT expressing C2C12 myotubes compared with control cells, suggesting that neither Wnt7a-CT nor Wnt7a-FL act through the canonical Wnt pathway. ( d ) Electroporation of a Wnt7a-CT or Wnt7a-FL expression plasmid into the TA muscle of C57/BL6 mice resulted in increased levels of pAKT compared with muscles electroporated with a control plasmid. Staining for HA in red, pAKT in green, laminin in white, nuclei are counterstained with Dapi (in blue). Electroporated fibres are marked by an asterisk. Scale bar: 20 μm. ( e ) Co-immunoprecipitation analysis demonstrates that both Wnt7a-CT and Wnt7a-FL bind Fzd7-YFP. ( f ) Co-immunoprecipitation analysis suggests that Wnt7a-CT and Wnt7a-FL bind to Fzd7-YFP with similar affinity. All P -values were calculated using a two-tailed Student’s t -test. All data are expressed as mean±s.e.m. Full size image We previously demonstrated that Wnt7a-FL binds to its receptor Fzd7 in myotubes [8] . To confirm that Wnt7a-CT also binds Fzd7, we performed a co-immunoprecipitation experiment. Briefly, we expressed either Wnt7a-CT (hemagglutinin (HA)-tagged) or Wnt7a-FL (HA)-tagged) together with Fzd7-YFP or YFP (control) and performed immunoprecipitations using green fluorescent protein (GFP)-antibody-coupled beads and immunoblot analysis for the HA-tag. Thereby, we demonstrated that Wnt7a-FL as well as Wnt7a-CT bind to Fzd7-YFP ( Fig. 3e ). To investigate the relative affinities of Wnt7a-CT and Wnt7a-FL binding to Fzd7, we performed a competition-based co-immunoprecipitation analysis ( Fig. 3f ). Briefly, varying amounts of Wnt7a-CT and Wnt7a-FL were co-expressed together with Fzd7-YFP. Immunoprecipitations were performed with GFP-antibody-coupled beads and immunoprecipitates subjected to immunoblot detection for the HA-tag that is present on both Wnt7a forms. When equivalent amounts of Wnt7a-CT and Wnt7a-FL are expressed together with Fzd7-YFP, we detected similar ratios of both full-length and C-terminal forms co-precipitating with Fzd7-YFP. Shifting the ratio of the amount of Wnt7a-CT to Wnt7a-FL expression in the direction of Wnt7a-CT resulted in more Wnt7a-CT detected in the precipitate and vice versa . Therefore, we conclude that Wnt7a-CT and Wnt7a-FL bind Fzd7-YFP with similar affinities. The activation of the AKT/mTOR pathway in myotubes and myofibres through Wnt7a is independent of GSK3beta and beta-catenin activation [8] . To demonstrate that Wnt7a-CT also acts non-canonically in this cellular context, we investigated the activation of these two members of the canonical Wnt signaling pathway. Indeed, Wnt7a-CT did not activate either GSK3beta or beta-catenin ( Fig. 3c , Supplementary Fig. S2 ), strongly supporting the assertion that Wnt7a-CT maintains its specificity for its receptor Fzd7 in skeletal muscle. We next investigated whether Wnt7a-CT can activate canonical Wnt signaling in other cell types as previously described for Wnt7a-FL [13] , [14] . Therefore, we assessed the activation of the beta-catenin gene reporter TopFlash in both Ishikawa cells and PC12 cells ( Fig. 4a,b ) as well as activation levels of GSK3beta and beta-catenin in PC12 cells ( Fig. 4c,d ). Notably, Wnt7a-CT activated the canonical Wnt signaling pathway in both cell types as demonstrated before for Wnt7a-FL. Therefore, we conclude that Wnt7a-CT is fully functional in different cell types maintaining its specificity and that palmitoylation is not required for activation of canonical or non-canonical Wnt7a signaling. 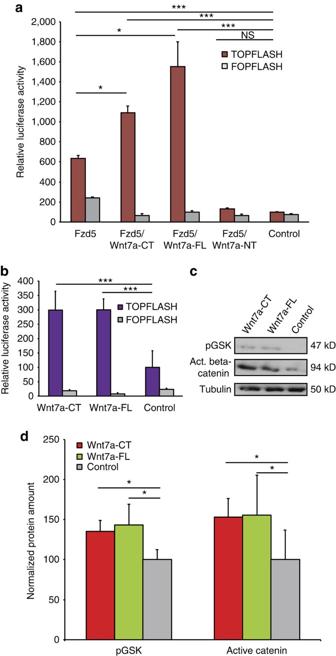Figure 4: Wnt7a-CT and Wnt7a-FL activate the canonical Wnt signaling pathway in Ishikawa and PC12 cells. (a) Cotransfection of Fzd5 and Wnt7a-CT or Wnt7a-FL into Ishikawa cells promotes significant activation of the beta-catenin TopFlash gene reporter. Luciferase activity was measured 24 h after transfection and normalized to protein amounts,n=4, *P<0.05, ***P<0.001. (b) Transfection of Wnt7a-CT or Wnt7a-FL into PC12 cells leads to activation of the beta-catenin TopFlash gene reporter. Luciferase activity was measured 24 h after transfection and normalized to protein amounts,n=4, ***P<0.001. (c) Immunoblot analyses revealed increased levels of phosphorylation of GSK3beta and activated beta-catenin in PC12 cells 48 h after transfection. (d) Densitometric analysis as inb(n=3), *P<0.05. AllP-values were calculated using a two-tailed Student’st-test. All data are expressed as mean±s.e.m. Figure 4: Wnt7a-CT and Wnt7a-FL activate the canonical Wnt signaling pathway in Ishikawa and PC12 cells. ( a ) Cotransfection of Fzd5 and Wnt7a-CT or Wnt7a-FL into Ishikawa cells promotes significant activation of the beta-catenin TopFlash gene reporter. Luciferase activity was measured 24 h after transfection and normalized to protein amounts, n =4, * P <0.05, *** P <0.001. ( b ) Transfection of Wnt7a-CT or Wnt7a-FL into PC12 cells leads to activation of the beta-catenin TopFlash gene reporter. Luciferase activity was measured 24 h after transfection and normalized to protein amounts, n =4, *** P <0.001. ( c ) Immunoblot analyses revealed increased levels of phosphorylation of GSK3beta and activated beta-catenin in PC12 cells 48 h after transfection. ( d ) Densitometric analysis as in b ( n =3), * P <0.05. All P -values were calculated using a two-tailed Student’s t -test. All data are expressed as mean±s.e.m. Full size image Wnt7a-CT stimulates symmetric satellite stem cell divisions Wnt7a drives the symmetric expansion of satellite stem cells by signalling through Fzd7 to activate the planar-cell polarity pathway, leading to a dramatic increase in the overall number of satellite cells as well as accelerated and augmented regeneration [7] . To investigate whether Wnt7a-CT also stimulates the symmetric expansion of satellite stem cells, we electroporated TA muscles with expression plasmids and enumerated the increase in numbers of satellite cells 3 weeks after electroporation. Muscles electroporated with the Wnt7a-CT expression plasmid showed a 57% increase in satellite cell numbers, whereas expression of Wnt7a-FL resulted in a 58% increase in the number of satellite cells ( Fig. 5a,b ). Furthermore, we injected cell culture supernatant containing either 150 ng of Wnt7a-CT or Wnt7a-FL protein into the TA muscle and quantified the numbers of satellite cells ( Fig. 5c ). Injection of supernatant containing equal amounts of Wnt7a-CT or Wnt7a-FL protein leads to a threefold increase in numbers of Pax7-positive satellite cells, whereas supernatant containing Wnt7a-NT protein did not have an effect on satellite cell numbers ( Fig. 2e ). These results indicate that Wnt7a-CT is fully capable of stimulating an increase in satellite cell numbers in vivo . 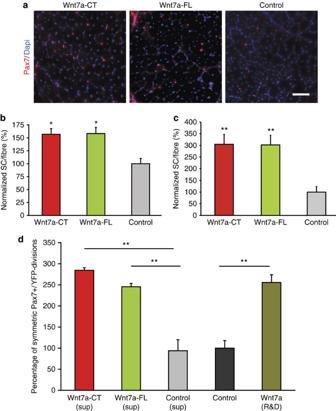Figure 5: Wnt7a-CT stimulates the expansion of the satellite stem cell pool. (a) Representative images of immunostained sections of TA muscles stained for Pax7 (in red); nuclei are counterstained with Dapi (in blue). Scale bar: 100 μm. (b) Electroporation of a Wnt7a-CT plasmid stimulates the expansion of satellite cells in TA muscles,n=4, *P<0.05. (c) Injection of Wnt7a-CT protein stimulates the expansion of satellite cells in TA muscles,n=4, **P<0.01. (d) Application of Wnt7a-CT stimulates the expansion of the satellite stem cell pool on single fibres after 42 h of culture,n=4, **P<0.01. AllP-values were calculated using a two-tailed Student’st-test. All data are expressed as mean±s.e.m. Figure 5: Wnt7a-CT stimulates the expansion of the satellite stem cell pool. ( a ) Representative images of immunostained sections of TA muscles stained for Pax7 (in red); nuclei are counterstained with Dapi (in blue). Scale bar: 100 μm. ( b ) Electroporation of a Wnt7a-CT plasmid stimulates the expansion of satellite cells in TA muscles, n =4, * P <0.05. ( c ) Injection of Wnt7a-CT protein stimulates the expansion of satellite cells in TA muscles, n =4, ** P <0.01. ( d ) Application of Wnt7a-CT stimulates the expansion of the satellite stem cell pool on single fibres after 42 h of culture, n =4, ** P <0.01. All P -values were calculated using a two-tailed Student’s t -test. All data are expressed as mean±s.e.m. Full size image Using Myf5-Cre and R26R-YFP reporter alleles, satellite stem cells, which have never expressed Myf5-Cre (Pax7 + /YFP − ), extensively contribute to the satellite cell pool after transplantation into muscle, whereas satellite myogenic cells, which express Myf5-Cre (Pax7 + /YFP + ), undergo terminal differentiation. Satellite stem cells can either undergo a symmetric planar cell division, or alternatively undergo an asymmetric apical-basal cell division to give rise to a satellite myogenic cell [15] . Wnt7a drives the symmetric expansion of satellite stem cells resulting in a dramatic increase in satellite cell number [7] . To investigate whether the activity of Wnt7a-CT is stimulating symmetric satellite stem cell divisions, isolated single myofibres from extensor digitorum longus (EDL) muscles of Myf5-Cre/R26R-YFP mice were cultured in the presence of medium containing Wnt7a-CT versus Wnt7a-FL for 42 h. Cultured myofibres incubated with Wnt7a-CT showed a 2.9-fold increase in symmetric satellite stem cell divisions, giving rise to two identical daughter stem cells. A similar increase in symmetric satellite stem cell divisions was observed following stimulation with the Wnt7a full-length protein (2.5-fold increase) ( Fig. 5d ). Therefore, we conclude that Wnt7a-CT is fully capable of driving the symmetric expansion of satellite stem cells in vitro and in vivo . Enhanced dispersal of Wnt7a-CT in tissue The amino-acid sequence of the C-terminus of Wnt7a suggests higher solubility in an aqueous solution than full-length Wnt7a. Therefore, to assess the dispersal of Wnt7a-CT in tissue, we electroporated TA muscles with low concentrations of Wnt7a-CT or Wnt7a-FL expression plasmids, such that <10% of all myofibres expressed the electroporated plasmid. Electroporated myofibres were visualized using immunostaining for the HA-tag present on all Wnt7a variants. We then measured the minimal fibre feret of the electroporated myofibre as well as the surrounding fibres. The surrounding myofibres were then binned into first, second or third order of myofibres ( Fig. 6b ). 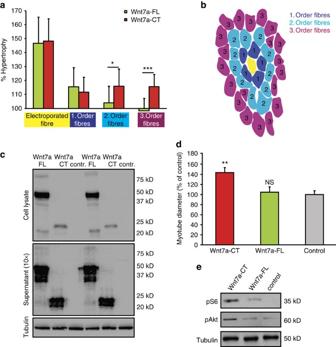Figure 6: Wnt7a-CT demonstrates increased dispersion compared with Wnt7a-FL. (a) Fibres surrounding a single fibre electroporated with a Wnt7a-CT expression plasmid show larger minimal fibre ferets at the second and third order when compared with fibres surrounding a single fibre electroporated with a Wnt7a-FL expression plasmid, the fibre feret was normalized to control electroporated fibres.n=4, ***P<0.001, *P<0.05. (b) Schematic showing the evaluation of fibre feret following electroporation of Wnt7a-CT or Wnt7a-FL. The electroporated fibre (marked by the expression of HA) is depicted in yellow. (c) COS cells transfected with a Wnt7a-CT expression plasmid show increased ratio of secreted protein to intracellular protein compared with Wnt7a-FL. Antibodies against HA were used to detect the truncated and full-length variant. (d) Transwell assay culturing COS cells either expressing Wnt7a-CT or Wnt7a-FL in the upper compartment and differentiating C2C12 cells on the lower compartment. Only C2C12 cells exposed to the supernatant from COS cells expressing the Wnt7a-CT variant demonstrate hypertrophy,n=4, **P<0.01. (e) Differentiated C2C12 cells exposed to the supernatant from COS cells using a transwell assay show increased amounts of phosphorylated (activated) S6 and AKT. AllP-values were calculated using a two-tailed Student’st-test. All data are expressed as mean±s.e.m. Figure 6: Wnt7a-CT demonstrates increased dispersion compared with Wnt7a-FL. ( a ) Fibres surrounding a single fibre electroporated with a Wnt7a-CT expression plasmid show larger minimal fibre ferets at the second and third order when compared with fibres surrounding a single fibre electroporated with a Wnt7a-FL expression plasmid, the fibre feret was normalized to control electroporated fibres. n =4, *** P <0.001, * P <0.05. ( b ) Schematic showing the evaluation of fibre feret following electroporation of Wnt7a-CT or Wnt7a-FL. The electroporated fibre (marked by the expression of HA) is depicted in yellow. ( c ) COS cells transfected with a Wnt7a-CT expression plasmid show increased ratio of secreted protein to intracellular protein compared with Wnt7a-FL. Antibodies against HA were used to detect the truncated and full-length variant. ( d ) Transwell assay culturing COS cells either expressing Wnt7a-CT or Wnt7a-FL in the upper compartment and differentiating C2C12 cells on the lower compartment. Only C2C12 cells exposed to the supernatant from COS cells expressing the Wnt7a-CT variant demonstrate hypertrophy, n =4, ** P <0.01. ( e ) Differentiated C2C12 cells exposed to the supernatant from COS cells using a transwell assay show increased amounts of phosphorylated (activated) S6 and AKT. All P -values were calculated using a two-tailed Student’s t -test. All data are expressed as mean±s.e.m. Full size image We did not observe any difference in the degree of hypertrophy of the myofibres electroporated with the Wnt7a-CT plasmid or Wnt7a-FL plasmids in the adjacent first-order fibres. However, Wnt7a-CT efficiently stimulated hypertrophy of second and third order, whereas Wnt7a-FL only stimulated hypertrophy in the first-order fibres and displayed little or no activity in the second or third order fibres ( Fig. 6a , Supplementary Fig. S3b ). Therefore, we conclude that Wnt7a-CT exhibits enhanced dispersal through muscle tissue. To investigate the efficiency of secretion of Wnt7a-CT, we transiently transfected COS cells with equal amounts of the different expression plasmids and assessed the amount of Wnt7a present in the supernatant relative to the cell lysate ( Fig. 6c ). We observed a marked increase in the ratio of supernatant to intracellular for Wnt7a-CT compared with Wnt7a-FL. Taken together, these data suggest that the Wnt7a-CT exhibits enhanced secretion relative to the full-length Wnt7a. Lastly, we used a transwell chamber assay to assess the dispersion of Wnt7a-CT compared with Wnt7-FL across a polycarbonate membrane. Briefly, we seeded C2C12 myoblasts on the bottom of the well and differentiated them for 3 days. COS cells either expressing the Wnt7a-CT or the Wnt7a-FL construct were added in the upper transwell chamber and incubated for two additional days. Only the myotubes exposed to the Wnt7a-CT variant demonstrated increased myotube diameters (1.4-fold, Fig. 6d , Supplementary Fig. S3a ) and increased levels of pAKT and pS6 ( Fig. 6e ). Therefore, Wnt7a-CT but not Wnt7a-FL can diffuse across the polycarbonate membrane. Together, these data indicate that the reduced size and absence of palmitoylation result in a protein with enhanced dispersal properties. Wnt proteins are promising candidates for therapeutic intervention. However, Wnt proteins are highly hydrophobic due to the addition of fatty acids. So far, all efforts to generate fully biologically active mammalian non-lipidated Wnt variants have failed [6] , [16] . Here we have demonstrated that truncated Wnt7a consisting of the C-terminal 137 aa and lacking palmitoylation sites is fully functional. Our results further suggest that the functionally active domain of Wnt7a is located in the C-terminus of the protein. Wnt7a-CT was able to fully activate the AKT/mTOR pathway and thereby induce hypertrophy, whereas the N-terminus of Wnt7a did not. The C-terminus of Wnt7a was also sufficient to stimulate divisions of satellite stem cells and bind to its receptor Fzd7 with similar affinity as the full-length protein ( Fig. 3e,f ) was also fully capable of stimulating the activation of canonical β-catenin/TCF signalling in PC12 and Ishikawa cells. Binding of Wnt7a-CT to Fzd7 is in accordance with a recent publication demonstrating that the C-terminal domain of XWnt8 makes close contacts with the Fzd8 receptor [12] . Janda et al. [12] found that XWnt8 made contact with Fzd8 at two points resembling a U-shaped clamp. From serine-187 of the N-terminus of XWNT8, a palmitoleic acid lipid group inserts into a deep groove in the cysteine-rich domain of Fz8, whereas the C-terminal portion of XWnt8 binds a hydrophobic depression on the opposite surface of the cysteine-rich domain. Our results suggest that the binding specificity exhibited by Wnt7a to its receptor Fzd7 is largely attributable to the C-terminal part of the protein. Although Janda et al. [12] had shown that the C-terminal part of XWnt8 binds to Fzd8, they did not demonstrate the functional outcome of this binding. Here we demonstrate that binding of the C-terminus of Wnt7a to Fzd7 leads to activation of the downstream pathways, resulting in either increased fibre feret or increased satellite stem cell numbers. Importantly, the Wnt7a-CT variant we generated exhibits enhanced dispersion and secretion relative to the full-length protein. Our work establishes for the first time that a mammalian non-palmitoylated truncated version of a Wnt protein is fully functional and opens important new avenues for the development of a Wnt7a-based biologic drug for the treatment of muscle-wasting disease. Electroporation and protein injections of TA muscles For in vivo electroporation, 40 μg of plasmid DNA (CMV-Wnt7a-FL-HA, CMV-Wnt7a-CT-HA or empty vector as control) in 0.9% NaCl was injected directly into the right TA muscle of anesthetized female C57BL/6 mice (10 weeks of age). Immediately after plasmid injection, electric stimulation was applied directly to the TA muscle using a pulse generator (ECM 830, BTX) of 100 volts for 6 pulses, with a fixed duration of 20 ms and an interval of 200 ms between the pulses equipped with a 5-mm needle electrode (BTX). Cell culture supernatant containing equal amounts of Wnt7a-FL-HA, Wnt7a-CT-HA or Wnt7a-NT-HA proteins were injected in a volume of 50 μl into the TA muscle of female C57/BL6 mice. For determination of protein concentration of the different Wnt7a variants, we performed immunoblots using antibodies directed to the HA-tag, which is present in all variants and/or antibodies directed to Wnt7a and quantified the grey values. Experimental and contralateral muscles were isolated and embedded in OCT-10%sucrose (Tissue-Tec) and cooled with liquid nitrogen. Cross-sections (14 μm) of the muscle were obtained using a cryostat (Leica CM1850). To ensure that the same areas of the muscles were compared, we cut the TA muscle in the middle of the belly and counted the sections, which were used for immunostainings. Mice were killed 2 weeks after electroporation or injection of culture supernatant containing the different Wnt7a variants. All experiments were performed following the regulations of the University of Ottawa for animal handling and animal care. Cell culture and transfection C2C12 myoblasts were cultured in DMEM with 20% fetal bovine serum (FBS) and were differentiated into myotubes in DMEM containing 2% horse serum [8] . C2C12 cells were transfected with the expression plasmids or siRNA (Ambion) using Lipofectamine 2000 (Roche) [17] . Transwell assays were carried out using the Transwell Permeable Supports 3.0 μm Polycarbonate Membrane system from Costar. Briefly, C2C12 cells were seeded in the lower compartment and differentiated for 3 days. On day 3 of differentiation, we added the upper compartment containing COS cells expressing the different Wnt7a variants. The TOPFLASH assay [18] was performed using the SuperTop vector system (Upstate) and a luciferase assay kit (Promega). PC12 or Ishikawa cells were transfected with expression plasmids for the different Wnt variants and a TOPflash vector containing TCF/LEF-binding sites followed by the luciferase gene. As a control we used a FOPflash vector containing mutated TCF/LEF-binding sites. PC12 cells were cultured in DMEM supplemented with 2 mmol l −1 glutamine and 10% FBS, whereas Ishikawa cells were grown in RPMI 1640 with glutamine and supplemented with 10% FBS, 0.01 mol l −1 HEPES [13] , [14] . EDL single fibre cultures EDL fibres were isolated through digestion with collagenase and cultured in DMEM supplemented with 20% FBS and 1% chick embryo extract [7] . Protein and RNA analyses Western blot, immunoprecipitation and immunofluorescence analyses were performed as described previously [19] . Immunoprecipitation was conducted using Chromotek-GFP-Trap beads purchased from Allele Biotechnology and Pharmaceuticals according to the instructions provided by the manufacturer. For immunofluorescence, cells or cryosections were fixed in ethanol (100%), incubation with primary antibodies was performed over night at 4 °C. Western blot analyses were conducted using polyvinylidene difluoride membranes (Immobilon), as blocking buffer we used 5% milk powder in TBS (1 × ). RNA extraction was conducted using the NucleoSpin II extraction kit from Machery-Nagel according to instructions provided by the manufacturer. Quantitative RT–PCR was performed using SYBR Green [7] . Antibodies used in this study are listed in Supplementary Table S1 , and the primers in Supplementary Table S2 . Full-length images of immunoblots are shown in Supplementary Fig. S4 . Wnt7a-CT-HA, Wnt7a-NT-HA and Wnt7a-FL-HA protein containing supernatant was generated by transfection of COS cells and concentration of the supernatant using Amicon Ultra-4 Centrifugal filters. Briefly, COS cells were transiently transfected with expression plasmids for the different Wnt7a variants using Lipofectamine 2000 (Roche) according to the instructions provided by the manufacturer. Two days after transfection, the culture supernatant was collected, and residual floating cells were removed through centrifugation. Afterwards, the supernatant was concentrated using Amicon Ultra-4 Centrifugal filters (10-kD cutoff) at 4 °C. The concentrated supernatant was aliquoted and stored at −20 °C. For determination of the concentration of the different Wnt7a variants, we performed immunoblots using antibodies directed to Wnt7a and/or HA and quantified the grey values. To exclude effects of the culture medium, we used concentrated supernatant from control cells to adjust injection volumes. Statistical analyses A minimum of three replicates were analysed for each experiment presented. Error bars are presented as standard error of the mean (Microsoft Excel), we assessed statistical significance using a two-tailed Student’s t -test (Microsoft Excel). Differences were considered as statistically significant with a P -value <0.05. How to cite this article: von Maltzahn, J. et al. A truncated Wnt7a retains full biological activity in skeletal muscle. Nat. Commun. 4:2869 doi: 10.1038/ncomms3869 (2013).